Lgr5+ cells regenerate hair cells via proliferation and direct transdifferentiation in damaged neonatal mouse utricle Recruitment of endogenous progenitors is critical during tissue repair. The inner ear utricle requires mechanosensory hair cells (HCs) to detect linear acceleration. After damage, non-mammalian utricles regenerate HCs via both proliferation and direct transdifferentiation. In adult mammals, limited transdifferentiation from unidentified progenitors occurs to regenerate extrastriolar Type II HCs. Here we show that HC damage in neonatal mouse utricle activates the Wnt target gene Lgr5 in striolar supporting cells. Lineage tracing and time-lapse microscopy reveal that Lgr5+ cells transdifferentiate into HC-like cells in vitro . In contrast to adults, HC ablation in neonatal utricles in vivo recruits Lgr5+ cells to regenerate striolar HCs through mitotic and transdifferentiation pathways. Both Type I and II HCs are regenerated, and regenerated HCs display stereocilia and synapses. Lastly, stabilized ß-catenin in Lgr5+ cells enhances mitotic activity and HC regeneration. Thus Lgr5 marks Wnt-regulated, damage-activated HC progenitors and may help uncover factors driving mammalian HC regeneration. Tissue injury activates endogenous stem/progenitor cells to regenerate lost cells, and disproportionate responses can result in disease states. The integumentary and intestinal systems are capable of self-renewing at baseline and after damage [1] , [2] , [3] , [4] , whereas the mature mammalian cochlea, which relies on sensory hair cells (HC) to detect auditory information, lacks the ability to regenerate new mechanoreceptive HCs. Within this spectrum of regenerative capacity is the mammalian utricle, a vestibular organ that requires HCs to detect linear acceleration and has a limited capacity to regenerate. In birds, both the basilar papilla (cochlea) and utricle robustly regenerate lost HCs [5] , [6] , [7] , [8] , [9] . This regenerative process consists of: (1) renewed/upregulated supporting cell (SC) proliferation and subsequent differentiation into HCs; and (2) phenotypic conversion, a mechanism termed direct transdifferentiation. In this mechanism, a SC converts into a HC without undergoing a mitotic division. After damage, these two processes (mitotic and non-mitotic regeneration) occur in distinct spatiotemporal patterns [10] , [11] . The utricle consists of two types of HCs (Type I and II or HC-I and HC-II), which are distinguished by morphology, ion channel composition, expression of calcium-binding proteins and synaptic innervation patterns [12] , [13] , [14] . HC-I’s reside predominantly in the J-shaped striolar region and HC-II’s in the extrastriolar region ( Supplementary Fig. 1 ). During regeneration of the avian utricle, both HC-I’s and HC-II’s are robustly replenished to restore vestibular function [7] , [15] . In contrast, the mammalian utricle regenerates only a small percentage of lost HCs in vitro and in vivo [16] , [17] , [18] , [19] , [20] , [21] , [22] , [23] , [24] , with little to no proliferation observed after HC loss [16] , [18] , [19] , [21] , [23] , [25] . Therefore, the primary mode of regeneration is assumed to be direct transdifferentiation. These replacement HCs appear to be exclusively of the Type II phenotype, and spontaneous regeneration of HC-I’s has not been reported in mammals [23] , [26] . Finally, regeneration occurs mainly in the extrastriolar region with the extent of recovery reaching only 18% at 6–8 months after damage [23] , [26] . Within the sensory epithelium, HCs are interdigitated by SCs. Several lines of evidence suggest that SCs are the sources of regenerated HCs. First, cells isolated from the sensory epithelium can behave as HC progenitors [27] , [28] . Second, a subset of SCs express the HC transcription factor Atoh1 after damage [18] , [23] . Third, SCs are occasionally labelled with mitotic tracers after damage [16] , [19] , [20] , [25] . However, a lineage marker of HC progenitors in the mammalian utricle has not been identified. Wnt signalling plays essential roles in the regulation of tissue homoeostasis by directing self-renewal of somatic stem cells [29] . Lgr5 is a Wnt target gene that marks somatic stem cells in self-regenerating organs [1] , [2] as well as progenitor cells recruited in the damaged liver and pancreas [30] , [31] . In some tissues, injury upregulates Wnt signalling, which in turn promotes repair [32] , [33] . However, overactive Wnt signalling also induces pathologic states by perturbing cellular differentiation and causing uncontrolled proliferation [34] , [35] . Such conflicting effects have also been found in the developing cochlea, where in vivo activation of Wnt signalling in Lgr5+ SCs induces proliferation and a failure of differentiation into HCs [36] , [37] . In contrast, the identical manipulation in Sox2+ SCs induces proliferation and limited ectopic HC formation [37] , [38] . At present, the roles of Wnt-responsive cells after damage and whether Wnt/ß-catenin signalling promotes HC regeneration in the utricle are unknown. Here we report the emergence of Lgr5+ SCs in the striolar region of the utricle after HC loss in vitro and in vivo . In both models of HC loss, lineage tracing demonstrated that Lgr5+ SCs can act as HC precursors with both HC-Is and HC-IIs regenerated in vivo . Furthermore, ß-catenin stabilization enhanced mitotic HC regeneration by Lgr5+ cells. Based on these data, we propose Lgr5+ SCs as damage-recruited Wnt-regulated HC progenitors in the mammalian utricle. Damage activates Lgr5 expression in supporting cells in vitro We examined utricles from neonatal Lgr5 EGFP-CreERT2/+ mice [1] , which report active Wnt signalling and Lgr5 expression in the cochlea [36] , [39] . In the cochlea, Lgr5-enhanced green fluorescent protein (Lgr5–EGFP) expression is regulated by Wnt signals, mirrors Lgr5 messenger RNA (mRNA) expression and persists into early adulthood [39] , [40] . In contrast, utricles from postnatal day 3 (P3) Lgr5 EGFP-CreERT2/+ mice demonstrated no detectable EGFP signal ( Fig. 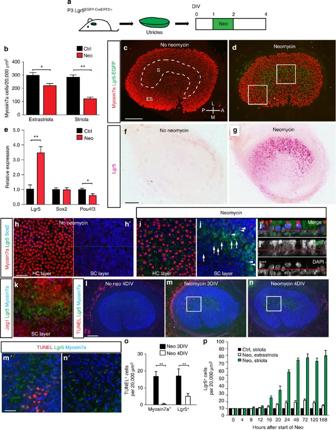Figure 1: Damage induces Lgr5 expressionin vitro. (a) Neomycin was used to damage hair cells (HCs) in utricles from P3Lgr5EGFP-CreERT2/+micein vitro. (b) Quantification of Myo7a+ HCs showed significant losses in striolar and extrastriolar regions. (c) Cultured, undamaged organs showed no Lgr5–EGFP signal. (d) Two days after neomycin treatment, Lgr5–EGFP was expressed in the striolar region, where HC loss was the most severe. (e) Quantitative PCR showed that damage caused a significant increase inLgr5mRNA expression, decrease inPou4f3expression, but no change inSox2expression. (f,g)In situhybridization showedLgr5mRNA transcripts in the striolar region of neomycin-treated utricles, whereas none were detected in cultured, undamaged organs. (h) Representative confocal images of undamaged, cultured utricles. (i–k) In damaged utricles, Lgr5+ cells expressed the SC markers Sox2 (arrowheads inj) and Jag1, but Sox2-negative Lgr5+ cells were also present (arrows). Lgr5+ cells rarely expressed Myo7a. The red line inj′–j′′′(side view) defines the boundary between the layers of HC and SC nuclei. (l–n) Unlike undamaged controls, neomycin-treated organs contained TUNEL+ cells in the striolar region 1 day post damage. (n) Lgr5+, TUNEL-negative cells were rare 2 days post damage. (o) TUNEL+/Myo7a+ and TUNEL+/Lgr5+ cells decreased in number post damage. (p) Lgr5+ cells rapidly increased in the striolar region after neomycin treatment and reached a plateau 48 h post damage.n=3 inb,e; 9 ini,j; 4 ink; 3–4 inl–oand 3 inp. Data shown as mean±s.d. *P<0.05, **P<0.01, Student’st-tests. Scale bars, (c,d,f,gandl–n) 100 μm; (h–kandm′–n′) 20 μm. 1c,h ) but had comparable HC densities and sensory epithelium dimensions to those of wild-type littermates ( Supplementary Table 1 ). Because mechanical damage to the sensory epithelium led to robust upregulation of Lgr5–EGFP ( Supplementary Fig. 1b ), we examined whether HC damage induces Lgr5 expression using a well-characterized paradigm of aminoglycoside-induced HC death (1.0 mM neomycin × 24 h, Fig. 1a ) [14] , [16] , [18] . This paradigm resulted in HC death preferentially in the striolar region ( Fig. 1b ), which is defined by oncomodulin expression in undamaged tissues ( Supplementary Fig. 1a ) [13] . Figure 1: Damage induces Lgr5 expression in vitro . ( a ) Neomycin was used to damage hair cells (HCs) in utricles from P3 Lgr5 EGFP-CreERT2/+ mice in vitro . ( b ) Quantification of Myo7a+ HCs showed significant losses in striolar and extrastriolar regions. ( c ) Cultured, undamaged organs showed no Lgr5–EGFP signal. ( d ) Two days after neomycin treatment, Lgr5–EGFP was expressed in the striolar region, where HC loss was the most severe. ( e ) Quantitative PCR showed that damage caused a significant increase in Lgr5 mRNA expression, decrease in Pou4f3 expression, but no change in Sox2 expression. ( f , g ) In situ hybridization showed Lgr5 mRNA transcripts in the striolar region of neomycin-treated utricles, whereas none were detected in cultured, undamaged organs. ( h ) Representative confocal images of undamaged, cultured utricles. ( i – k ) In damaged utricles, Lgr5+ cells expressed the SC markers Sox2 (arrowheads in j ) and Jag1, but Sox2-negative Lgr5+ cells were also present (arrows). Lgr5+ cells rarely expressed Myo7a. The red line in j′ – j′′′ (side view) defines the boundary between the layers of HC and SC nuclei. ( l – n ) Unlike undamaged controls, neomycin-treated organs contained TUNEL+ cells in the striolar region 1 day post damage. ( n ) Lgr5+, TUNEL-negative cells were rare 2 days post damage. ( o ) TUNEL+/Myo7a+ and TUNEL+/Lgr5+ cells decreased in number post damage. ( p ) Lgr5+ cells rapidly increased in the striolar region after neomycin treatment and reached a plateau 48 h post damage. n =3 in b , e ; 9 in i , j ; 4 in k ; 3–4 in l – o and 3 in p . Data shown as mean±s.d. * P <0.05, ** P <0.01, Student’s t -tests. Scale bars, ( c , d , f , g and l – n ) 100 μm; ( h – k and m′ – n′ ) 20 μm. Full size image Two days after neomycin treatment, many Lgr5–EGFP+ cells occupied the SC layer in the striolar region, whereas only a few were found in the extrastriolar region ( Fig. 1d , Supplementary Fig. 1j,u ). 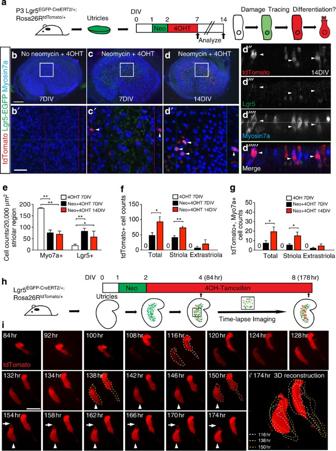Figure 2: Lgr5+ cells act as striolar hair cell precursorsin vitro. (a) Utricles from P3Lgr5EGFP-CreERT2/+; Rosa26RtdTomato/+mice were treated with neomycin and then 4OH-tamoxifen (4OHT) to fate-map Lgr5+ cells. Organs were examined after 7 or 14 daysin vitro(DIV). (b–b′) Undamaged controls had no tdTomato+ cells. (c-c′) Rare tdTomato+/Myo7a+ hair cells (HCs, arrowheads) were detected 7 days after damage, and (d–d′) many more double-labelled cells were found at 14DIV. (d″–d′′′′′) Orthogonal (XZ) views ofd′. (e) Neomycin caused significant loss of striolar HCs and an increase in Lgr5+ cells. (f,g) Both total tdTomato+ cells and tdTomato+/Myo7a+ cells significantly increased over time. (h) Schematic for time-lapse imaging of lineage-traced Lgr5+ cells over 94 h. (i) Stills of time-lapse (Supplementary Movie 1) capturing two tdTomato+ cells selected from Lgr5–EGFP+ cells. tdTomato signal was first present in the right cell and later appeared in the left cell. Both cells first appeared tall and slender and resembled supporting cells. The left cell gradually became flask shaped, beginning at 138 h (arrowhead indicates hair cell-like cell). The basolateral portion of the left cell rounds up and an apical protrusion appeared around 154 h (arrows). (i′) represents a three-dimensional reconstruction of images at 174 h. Dashed lines depict outlines of cells from stated time points.n=3–6 ine–g. Data are shown as mean±s.d. *P<0.05, **P<0.01, Student’st-tests. Scale bars, (b–d) 100 μm; (b′–d′) 20 μm; (i) 10 μm. We measured the dimension and location of the oncomodulin+ striolar region before damage and of Lgr5–EGFP+ domains after neomycin damage and found no significant differences ( Supplementary Table 2 ); we thus refer the Lgr5–EGFP+ domain as striolar. In situ hybridization showed Lgr5 mRNA expression in the striolar region 2 days after neomycin treatment but not in undamaged control tissues ( Fig. 1f,g ), thus corroborating spatiotemporal expression pattern of the Lgr5 –EGFP reporter mice. Longitudinal analyses revealed that Lgr5+ cells first appeared after 4 h of neomycin treatment, subsequently increased in number and remained predominantly in the striolar region ( Fig. 1p , Supplementary Fig. 1c–m ). In the extrastriolar region where damage was less severe, rare Lgr5+ cells were transiently detected ( Fig. 1p , Supplementary Fig. 1n–x ). Twenty-four hours after damage, occasional Myo7a+ and Lgr5+ cells were stained by terminal deoxynucleotidyl transferase dUTP nick end labelling (TUNEL; Fig. 1m ), indicating degenerating cells. While dying Myo7a+ and Lgr5+ cells significantly decreased 48 h post damage ( Fig. 1l,m ); the number of Lgr5+ cells increased and reached a plateau between 48 and 72 h and remained robust for at least 6 days post damage ( Fig. 1p , Supplementary Fig. 1c–m ). At all time points examined, Lgr5+ cells resided in the SC layer ( Fig. 1i–k ). Jag1 and Sox2 are both expressed in SCs with the latter also marking Type II HCs. Immunostaining 48 h after neomycin treatment showed that all Lgr5+ cells expressed Jag1 ( n =4), but only a subset of them expressed Sox2 (26.9±38.2%, n =9, Fig. 1i–k ). Lgr5+ cells occasionally expressed the HC markers Gfi1 (3.2±1.9%) and Myo7a (2.5±1.3%), but never the proliferation marker Ki67 ( Fig. 1i–k , Supplementary Fig. 6a–c , Supplementary Table 6 ). To validate and quantify Lgr5 expression after damage, we measured Lgr5 mRNA levels in utricles from P3 wild-type mice identically damaged by neomycin in vitro . In comparison to non-damaged, cultured controls, Lgr5 mRNA expression tripled in neomycin-treated cultures ( P <0.01, Student’s t -test), whereas Pou4f3 decreased significantly ( P <0.05, Student’s t -test) and Sox2 expression did not significantly change ( Fig. 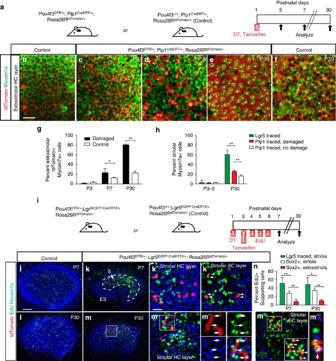Figure 6: Striolar and extrastriolar supporting cells behave differently after damage. (a) Schematic depicting the use of transgenic mice to ablate hair cells (HCs) and fate-map Plp1+ supporting cells (SCs). (b,c) Tamoxifen led to tdTomato labelling of extrastriolar SCs at P3 (also seeSupplementary Fig. 4). (d–f) In both P7 undamaged (not shown) and damaged organs, a subset of Myo7a+ HCs were tdTomato+ (asterisks). Most extrastriolar HCs were tdTomato+ in the P30 damaged utricles, whereas only a subset of HCs were tdTomato+ in the P30 undamaged controls (f). (g) Quantification showed that damaged organs had significantly more lineage-traced HCs than undamaged controls in the extrastriolar region at P7 and P30 (n=520–1,884 cells from 4–6 organs). (h) In the striolar region where Lgr5 was expressed after damage, significantly more HCs derived from the Lgr5+ than Plp1+ lineage (n=635 from 28 organs and 1,232 cells from 4 organs, respectively). (i) Schematic showing the use of transgenic mice to ablate HCs and fate-map Lgr5+ striolar SCs, and EdU to trace dividing cells. (j–m) Undamaged utricles contained few EdU-labelled cells in the sensory epithelium. Damage caused robust EdU labelling in the striolar region, where lineage-traced Lgr5+ cells resided. At P7, most EdU+ cells were Myo7a negative and resided in the SC layer, including EdU+, lineage-traced cells (arrowheads). At P30, many EdU+/tdTomato+/Myo7a+ HCs (arrowheads) were present. (m′′′) Many EdU+/tdTomato+/Myo7a-negative SCs were also found at P30 (arrows). (m′′′′) shows an orthogonal view ofm′(n=602 cells from 6 organs). (n) Quantification of EdU labelling showed that the Lgr5+ lineage (Myo7a-negative SCs in (m′′′) was more proliferative than Sox2+ SCs in the striolar and extrastriolar regions (seeSupplementary Fig. 5c,e).n=4–8 ingandn, and 4–28 inh(4–8 for P3–5, 28 for Lgr5-traced P30 organs and 4–6 for Plp1-traced P30 organs). Data shown as mean±s.d. *P<0.05, **P<0.01, Student’st-tests. Scale bars, (b–f,j–m) 100 μm; (k′,k″,m′,m′′′) 20 μm. 1e ). The increase in Lgr5 transcripts in damaged wild-type organs is consistent with Lgr5 mRNA detected by in situ hybridization and also with the increased EGFP signal in damaged utricles from neonatal Lgr5 –EGFP reporter mice. Damage-activated Lgr5+ SCs generate HC-like cells in vitro Prior studies on adult utricles have demonstrated regenerated HCs after aminoglycoside-induced HC loss in vitro ; however, almost no proliferation has been observed [16] , [18] , [20] . Here we allowed neomycin-damaged neonatal utricles from P3 Lgr5 EGFP-CreERT2/+ mice to recover in aminoglycoside-free media for 5 or 12 days and did not detect any significant increase in the number of Myo7a+ HCs ( Fig. 2e ). Addition of the thymidine analogue EdU (1 μM × 5 days) failed to label Lgr5+ or Myo7a+ cells ( Supplementary Table 6 ), indicating that Lgr5+ cells were not proliferative in vitro . We then used lineage tracing to determine whether damage-activated Lgr5+ cells can act as precursors for regenerated HCs observed in prior studies. After utricles from P3 Lgr5 EGFP-CreERT2/+ ; Rosa26R tdTomato/+ mice [41] were damaged with neomycin, 4OH-tamoxifen (500 nM × 5 days) was added to aminoglycoside-free media to prospectively follow damage-induced Lgr5+ cells ( Fig. 2a ). In this model, tamoxifen-induced activation of Cre recombinase results in permanent labelling (tdTomato) of Lgr5+ cells and their progeny. Two days after neomycin-induced damage (48 h of 4OH-tamoxifen), few tdTomato-positive, Lgr5 lineage-traced cells were observed, none of which expressed Myo7a ( Supplementary Fig. 2a ). By 5 days after neomycin-induced damage, few cells expressed tdTomato and Myo7a. One week later (12 days after damage), the number of tdTomato+/Myo7a+ cells increased by 2.6-fold ( P <0.05, Student’s t -test, 7.3±2.5 cells and 19.3±5.0 cells at 7DIV and 14DIV, respectively, Fig. 2c,d,g ). These findings suggest that Lgr5+ SCs recruited after HC loss can contribute to the regeneration of HC-like cells in vitro . Addition of EdU (1 μM × 5 days) during the post-damage period did not label any tdTomato+/Myo7a+ cells ( Supplementary Table 6 ), suggesting that Lgr5+ SCs acquired a HC fate directly without undergoing mitosis. Figure 2: Lgr5+ cells act as striolar hair cell precursors in vitro . ( a ) Utricles from P3 Lgr5 EGFP-CreERT2/+ ; Rosa26R tdTomato/+ mice were treated with neomycin and then 4OH-tamoxifen (4OHT) to fate-map Lgr5+ cells. Organs were examined after 7 or 14 days in vitro (DIV). ( b – b′ ) Undamaged controls had no tdTomato+ cells. ( c - c′ ) Rare tdTomato+/Myo7a+ hair cells (HCs, arrowheads) were detected 7 days after damage, and ( d – d′ ) many more double-labelled cells were found at 14DIV. ( d″ – d′′′′′ ) Orthogonal (XZ) views of d′ . ( e ) Neomycin caused significant loss of striolar HCs and an increase in Lgr5+ cells. ( f , g ) Both total tdTomato+ cells and tdTomato+/Myo7a+ cells significantly increased over time. ( h ) Schematic for time-lapse imaging of lineage-traced Lgr5+ cells over 94 h. ( i ) Stills of time-lapse ( Supplementary Movie 1 ) capturing two tdTomato+ cells selected from Lgr5–EGFP+ cells. tdTomato signal was first present in the right cell and later appeared in the left cell. Both cells first appeared tall and slender and resembled supporting cells. The left cell gradually became flask shaped, beginning at 138 h (arrowhead indicates hair cell-like cell). The basolateral portion of the left cell rounds up and an apical protrusion appeared around 154 h (arrows). ( i′ ) represents a three-dimensional reconstruction of images at 174 h. Dashed lines depict outlines of cells from stated time points. n =3–6 in e – g . Data are shown as mean±s.d. * P <0.05, ** P <0.01, Student’s t -tests. Scale bars, ( b – d ) 100 μm; ( b′ – d′ ) 20 μm; ( i ) 10 μm. Full size image To further examine whether damage-recruited Lgr5+ cells undergo direct transdifferentiation, we performed time-lapse imaging concurrent with lineage tracing of damage-recruited Lgr5+ cells. As before, utricles from P3–5 Lgr5 EGFP-CreERT2/+ ; Rosa26R tdTomato/+ mice were first cultured and damaged with neomycin, then exposed to 4OH-tamoxifen to initiate labelling of Lgr5+ cells. Imaging began 2–4 days after damage and continued for 45–97 h ( Fig. 2h , Supplementary Fig. 2b ). Utricular HCs and SCs are morphologically distinct with HCs being shorter, round-bottomed and crowned apically with prominent stereocilia, while SCs are taller and narrower than HCs. Using these morphologic criteria, we analyzed time-lapse videos of 34 tdTomato+ cells (fate mapped from the Lgr5+ lineage) from four utricles. We observed 2 tdTomato-labelled lineage-traced cells that appeared to convert into HC-like cells ( Fig. 2i , Supplementary Fig. 2c–d , Supplementary Movies 1–3 ). After fixation, we also detected Myo7a expression in a subset of tdTomato+ cells ( Supplementary Fig. 2e ). Together these data indicate that damage-activated Lgr5+ SCs can act as HC precursors in vitro . Embryonic Lgr5+ cells contribute to reactivated Lgr5+ cells To determine the source of damage-activated Lgr5+ cells, we examined the embryonic utricle. Utricle development in mice begins around embryonic day 11.5 (E11.5) and extends into the first two postnatal weeks [42] , [43] , [44] . Prior to birth, 49% of HCs are present, and the sensory epithelium reaches 81% of its adult size [42] . Utricles from E15.5 Lgr5 EGFP-CreERT2/+ mice showed robust Lgr5–EGFP expression in the central region of the sensory epithelium and the EGFP+ cells more commonly expressed Sox2 than Myo7a (84.1±24.7% and 15.2±5.5%, respectively, n =428 cells from four organs, Fig. 3a ). Between E15.5 and P3, both Lgr5–EGFP+ cell counts and mRNA levels significantly decreased ( P <0.01, Student’s t -test, Fig. 3a–f ). At P3 and later ages, Lgr5–EGFP+ cells were undetectable ( n =3, Fig. 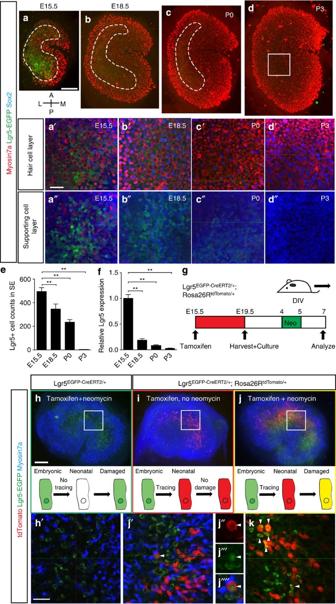3d,e ). Figure 3: Damage-induced Lgr5+ cells derive from embryonic Lgr5+ cells. (a–d) Representative images of utricle whole mounts from E15.5, 18.5, P0 and P3Lgr5EGFP-CreERT2/+mice. At E15.5, robust Lgr5–EGFP signals occupied most of the sensory epithelium, decreasing in intensity and proportion with age as the organ enlarges. (a′–d″) High magnification images showed EGFP signals in Sox2+ SCs and Myo7a+ hair cells, both decreasing with age. Inset positions shown ina–d. (e) Quantification of Lgr5–EGFP+ cells in sensory epithelia. (f) Quantitative PCR showed a significant decrease inLgr5mRNA expression with age. (g) Schematic for fate-mapping of E15.5 Lgr5+ cells. Tamoxifen was administered to dams, embryos from which were harvested at E19.5, and their utricles were cultured and damaged with neomycin. (h–h′) Control tissues (Lgr5EGFP-CreERT2/+) treated with tamoxifen and neomycin show Lgr5–EGFP+ SCs without tdTomato labelling. (i) Tamoxifen treatment without damage led to tdTomato labelling without Lgr5–EGFP signals. (j–j′′′) Tamoxifen treatment and damage resulted in a tdTomato+/Lgr5–EGFP+/Myo7a-negative cell (arrowhead). (k) Image of a separate utricle showing multiple tdTomato+/Lgr5–EGFP+ cells (arrowheads).n=3–5 ina–f. Data are shown as mean±s.d. **P<0.01, Student’st-tests. Scale bars, (a–d,h–j) 100 μm; (a′–d″,h′,j′andk) 20 μm. Figure 3: Damage-induced Lgr5+ cells derive from embryonic Lgr5+ cells. ( a–d ) Representative images of utricle whole mounts from E15.5, 18.5, P0 and P3 Lgr5 EGFP-CreERT2/+ mice. At E15.5, robust Lgr5–EGFP signals occupied most of the sensory epithelium, decreasing in intensity and proportion with age as the organ enlarges. ( a′ – d″ ) High magnification images showed EGFP signals in Sox2+ SCs and Myo7a+ hair cells, both decreasing with age. Inset positions shown in a – d . ( e ) Quantification of Lgr5–EGFP+ cells in sensory epithelia. ( f ) Quantitative PCR showed a significant decrease in Lgr5 mRNA expression with age. ( g ) Schematic for fate-mapping of E15.5 Lgr5+ cells. Tamoxifen was administered to dams, embryos from which were harvested at E19.5, and their utricles were cultured and damaged with neomycin. ( h – h′ ) Control tissues ( Lgr5 EGFP-CreERT2/+ ) treated with tamoxifen and neomycin show Lgr5–EGFP+ SCs without tdTomato labelling. ( i ) Tamoxifen treatment without damage led to tdTomato labelling without Lgr5–EGFP signals. ( j – j′′′ ) Tamoxifen treatment and damage resulted in a tdTomato+/Lgr5–EGFP+/Myo7a-negative cell (arrowhead). ( k ) Image of a separate utricle showing multiple tdTomato+/Lgr5–EGFP+ cells (arrowheads). n =3–5 in a – f . Data are shown as mean±s.d. ** P <0.01, Student’s t -tests. Scale bars, ( a – d , h – j ) 100 μm; ( a′ – d″ , h′ , j′ and k ) 20 μm. Full size image To determine the relationship between embryonic Lgr5+ cells and those re-expressing Lgr5 in response to HC loss, we performed lineage tracing in Lgr5 EGFP-CreERT2/+ ; Rosa26R tdTomato/+ mice. When tamoxifen was administered at E15.5, and the utricles were viewed at E19.5, a small number of both HCs and SCs in the striolar region expressed tdTomato (4.6±1.4% Myo7a+ and 6.0±1.1% Sox2+ cells, n =1,532–3,184 cells from 3 organs). Next we harvested utricles at E19.5 and cultured them for 4 days (equivalent to P3) before damaging them with neomycin ( Fig. 3g ). In control undamaged organs, lineage-traced cells (tdTomato+) but no Lgr5–EGFP+ cells were detected ( Fig. 3i ). Neomycin-treated utricles contained Lgr5–EGFP+ cells in the striolar region at 7DIV, a subset of which (29.4±35.7%, n =479 cells from 8 utricles) were tdTomato+ ( Fig. 3j,k ), indicating that they derived from embryonic Lgr5+ cells. In vivo HC ablation in Pou4f3 DTR/+ mice To investigate whether Lgr5+ cells can act as HC precursors after damage in vivo , we utilized Pou4f3-DTR mice [23] . In this mouse strain, the HC promoter Pou4f3 drives expression of the human diphtheria toxin receptor (DTR), thereby allowing selective HC ablation that can be temporally controlled by DT administration [23] , [45] , [46] . In P1 mice, a single DT injection (6.25 ng g −1 , i.p.) results in HC loss 2 days later ( Fig. 4a ). In contrast to the rapid HC loss centred in the striolar region caused by neomycin treatment in vitro , DT administration produced gradual HC loss encompassing the entire sensory epithelium. In comparison to age-matched control animals (wild-type littermates injected with DT), utricles from P3 Pou4f3 DTR/+ mice showed comparable reductions in HC densities in the striolar and extrastriolar regions ( Fig. 4b–k , Supplementary Fig. 3f,j , Supplementary Table 3 ). This degeneration was compounded by an overall decrease in the sensory epithelium (Myo7a+) area ( Fig. 4j , Supplementary Table 3 ). Over the next 12 days, both the HC number and the total area of the sensory epithelium decreased and reached their lowest points between P7 and P15 ( Fig. 4j,k , Supplementary Fig. 3n , Supplementary Table 3 ). The nadir of HC number of all time points (P3-30) examined was P15, at which point the striolar and extrastriolar HC densities were 29.1±20.5% and 24.5±17.4% of age-matched controls, respectively ( Fig. 4k , Supplementary Fig. 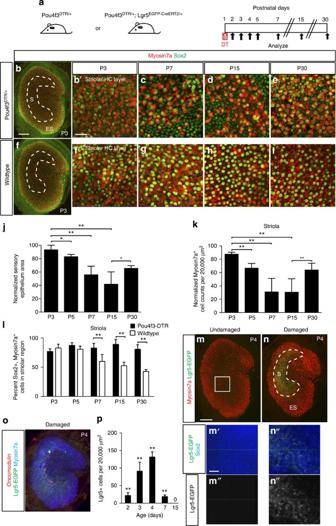3n ). Figure 4: Lgr5+ supporting cells emerge after hair cell ablationin vivo. (a) Schematic depicting the use of diphtheria toxin (DT) to ablate hair cells (HCs) inPou4f3DTR/+mice andLgr5EGFP-CreERT2/+mice to report Lgr5 expression. (b–e) DT treatment at P1 caused progressive HC loss and organ shrinkage over a 2-week period, followed by a partial recovery at P30. (f–i) Undamaged control organs from P3–P30. (j) Relative to age-matched, undamaged organs, DT-damaged organs were smaller. Damaged organs were the smallest at P15 and partly re-expanded at P30. (k) Normalized Myo7a+ cell counts similarly decreased and were the lowest at P15, before significantly increasing at P30 (P<0.0001, Student’st-test). (l) Quantification showed that the damaged organs fromPou4f3-DTRmice contained higher percentages of Sox2+/Myo7a+ cells than age-matched, undamaged organs at P7, P15 and P30. (m) No detectable Lgr5–EGFP signals in undamaged organs at P4. (n) DT-mediated HC loss led to robust Lgr5–EGFP expression in striolar Sox2+ supporting cells (SCs) at P4 (also seeSupplementary Fig. 3). 94.2±4.9% of Lgr5–EGFP+ SCs expressed Sox2+. (o) Lgr5–EGFP+ domain overlapped with the striola, where residual oncomodulin+ HCs resided. (p) Relative to age-matched, undamaged controls (Supplementary Fig. 3), there were significantly more Lgr5–EGFP+ cells after HC ablation P2–7 (P<0.01, Student’st-test).n=4–12 inj–l(4 for P3, 8 for P5 and 12 for P7, P15 and P30) and 4–6 inp. Data are shown as mean±s.d. *P<0.05, **P<0.01, Student’st-tests. Scale bars, (b,f,m–o) 100 μm; (b′,c–e,f′,g–i,m′–n″) 20 μm. Figure 4: Lgr5+ supporting cells emerge after hair cell ablation in vivo . ( a ) Schematic depicting the use of diphtheria toxin (DT) to ablate hair cells (HCs) in Pou4f3 DTR/+ mice and Lgr5 EGFP-CreERT2/+ mice to report Lgr5 expression. ( b – e ) DT treatment at P1 caused progressive HC loss and organ shrinkage over a 2-week period, followed by a partial recovery at P30. ( f – i ) Undamaged control organs from P3–P30. ( j ) Relative to age-matched, undamaged organs, DT-damaged organs were smaller. Damaged organs were the smallest at P15 and partly re-expanded at P30. ( k ) Normalized Myo7a+ cell counts similarly decreased and were the lowest at P15, before significantly increasing at P30 ( P <0.0001, Student’s t -test). ( l ) Quantification showed that the damaged organs from Pou4f3-DTR mice contained higher percentages of Sox2+/Myo7a+ cells than age-matched, undamaged organs at P7, P15 and P30. ( m ) No detectable Lgr5–EGFP signals in undamaged organs at P4. ( n ) DT-mediated HC loss led to robust Lgr5–EGFP expression in striolar Sox2+ supporting cells (SCs) at P4 (also see Supplementary Fig. 3 ). 94.2±4.9% of Lgr5–EGFP+ SCs expressed Sox2+. ( o ) Lgr5–EGFP+ domain overlapped with the striola, where residual oncomodulin+ HCs resided. ( p ) Relative to age-matched, undamaged controls ( Supplementary Fig. 3 ), there were significantly more Lgr5–EGFP+ cells after HC ablation P2–7 ( P <0.01, Student’s t -test). n =4–12 in j – l (4 for P3, 8 for P5 and 12 for P7, P15 and P30) and 4–6 in p . Data are shown as mean±s.d. * P <0.05, ** P <0.01, Student’s t -tests. Scale bars, ( b , f , m – o ) 100 μm; ( b′ , c – e , f′ , g – i , m′ – n″ ) 20 μm. Full size image In comparison to P15, both the number of HCs and the area of the sensory epithelium area had significantly (but incompletely) recovered by P30 ( Fig. 4j,k , Supplementary Fig. 3c–d,h–i,l–n , Supplementary Table 3 ). In undamaged utricles from P30 wild-type mice, 42.6±3.5% of striolar Myo7a+ HCs ( n =2,121 cells from 12 organs, Fig. 4l , Supplementary Fig. 3e ) expressed Sox2 and were classified as Type II (refs 23 , 47 ). However, more HCs in damaged utricles from P30 Pou4f3 DTR/+ mice expressed Sox2 (80.7±7.6%, P <0.0001, Student’s t -test, n =1,678 cells from 12 organs), suggesting that regenerated HCs were predominantly Type II. Our data using the Pou4f3 DTR/+ mice indicate that the neonatal mouse utricle spontaneously regenerates HCs in vivo . To investigate whether in vivo HC ablation also activates Lgr5 expression in SCs, we examined Lgr5 EGFP-CreERT2/+ ; Pou4f3 DTR/+ mice. After DT treatment at P1, Lgr5+ cells appeared 1 day later and increased in the subsequent 2 days ( Fig. 4p , Supplementary Fig. 3o–q ). At P4, Lgr5+ cells resided in the SC layer distributed in a striolar pattern and primarily expressed the SC marker Sox2 ( Fig. 4n′ ). The dimensions and location of Lgr5–EGFP domain after DT-mediated damage in vivo was not different from that of oncomodulin+ striolar region in age-matched, undamaged control utricles. At P4, the Lgr5–EGFP domain surrounded the remaining oncomodulin+ striolar HCs ( Fig. 4o ). Lgr5+ cells were rare at P7 and undetectable at P15 ( Fig. 4p , Supplementary Fig. 3r–s ). Thus similar to our findings in the in vitro preparation, these data indicate that in vivo HC ablation also reactivates Lgr5 in striolar SCs and led us to next determine their cell fate via lineage tracing. Damage-activated Lgr5+ SCs regenerate HC-like cells in vivo While most damage-recruited Lgr5+ cells did not express Myo7a (97.5±1.1%, P4), a significant portion expressed the early HC marker Gfi1 (21.2±5.7%, Supplementary Fig. 6e , Supplementary Table 6 ). Most Lgr5+ cells that were Gfi1+/Myo7a− were found in the supporting cell layer ( Supplementary Fig. 6e ). To determine the significance of this, we fate mapped Lgr5+ cells in Pou4f3 DTR/+ ; Lgr5 EGFP-CreERT2/+ ; Rosa26R tdTomato/+ mice. After DT was injected at P1 to initiate HC degeneration, tamoxifen was administered at P3 to lineage-trace Lgr5+ cells ( Fig. 5a ). At P4, 18.9±4.7% of Sox2+ SCs expressed Lgr5 after damage ( n =1,866 cells from 4 organs, Supplementary Fig. 3q ). Two days after tamoxifen treatment, occasional tdTomato-expressing SCs and few Myo7a+ HCs were traced ( Fig. 5c,f,g , Supplementary Table 4 ). In parallel controls ( Pou4f3 +/+ ; Lgr5 EGFP-CreERT2/+ ; Rosa26R tdTomato/+ identically administered with DT at P1 and tamoxifen at P3), no Lgr5–EGFP+ cells and only rare tdTomato+ cells were found ( Fig. 5b,f,g , Supplementary Fig. 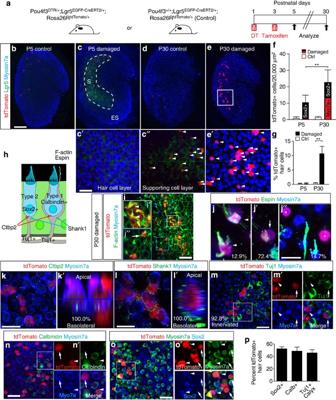4b–c , Supplementary Table 4 ). Figure 5: Lgr5+ cells act as hair cell progenitorsin vivo. (a) Schematic of the genetic approach to ablate hair cells and fate-map Lgr5+ cellsin vivo. (b) In undamaged tissues, Lgr5–EGFP signal was absent and tamoxifen rarely induced tdTomato labelling at P5. (c) By contrast, damaged utricles showed many tdTomato+/Lgr5+/Myo7a-negative cells (arrowheads inc′–c″) at P5. (d) Undamaged organs showed rare tdTomato labelling at P30. (e) P30 damaged utricles had many tdTomato+/Myo7a+ cells (arrowheads). (f) Relative to P5, P30 had significantly more tdTomato+ and tdTomato+/Myo7a+ cells. At P5, almost all tdTomato+ cells were Myo7a negative, whereas 60.6% expressed Myo7a at P30. (g) About 11% of striolar Myo7a+ hair cells (HCs) were tdTomato+ at P30. (h) Diagram illustrating Type I and II HCs. (i) Representative confocal images of P30 damaged and lineage-traced utricles, which contained tdTomato+/Myo7a+ cells with actin-enriched, bundle-like structures. (i′–i″) Lineage-traced HCs with long (arrowheads) and short stereocilia (arrow). (j–j″) Lineage-traced HCs showed long (j), and short (j′) espin+ stereocilia or were espin negative and bundleless (j″, labelled by asterisks). (k) All tdTomato+/Myo7a+ cells examined expressed Ctbp2 on the basolateral surfaces.k′shows an orthogonal view ofk. (l) Lineage-traced HCs were also juxtaposed to the postsynaptic protein Shank1.l′shows an orthogonal view ofl. (m–m′) 92.8% of lineage-traced HCs were innervated by Tuj1+ neurites (arrowhead), a subset of which formed calyces (arrows). (n) Lineage-traced HCs were calbindin negative (arrow) and positive (arrowhead). (o–o′) Lineage-traced, Myo7a+ HCs were Sox2 positive (arrowheads) and negative (arrows). (p) Quantification of lineage-traced HCs showed that about half were Sox2 negative (n=28 cells from 3 organs), calbindin positive (n=47 cells from 3 organs) and surrounded by Tuj1+ calyces (asterisk) (n=37 cells from 3 organs).n=4–5 at P5, 26–28 inf,g. Data are shown as mean±s.d. **P<0.01, Student’st-tests. Scale bars, (b–e) 100 μm; (c′–e′,i,m–o) 20 μm; (k) 10 μm; (i–j″,l) 5 μm. Figure 5: Lgr5+ cells act as hair cell progenitors in vivo . ( a ) Schematic of the genetic approach to ablate hair cells and fate-map Lgr5+ cells in vivo . ( b ) In undamaged tissues, Lgr5–EGFP signal was absent and tamoxifen rarely induced tdTomato labelling at P5. ( c ) By contrast, damaged utricles showed many tdTomato+/Lgr5+/Myo7a-negative cells (arrowheads in c′ – c″ ) at P5. ( d ) Undamaged organs showed rare tdTomato labelling at P30. ( e ) P30 damaged utricles had many tdTomato+/Myo7a+ cells (arrowheads). ( f ) Relative to P5, P30 had significantly more tdTomato+ and tdTomato+/Myo7a+ cells. At P5, almost all tdTomato+ cells were Myo7a negative, whereas 60.6% expressed Myo7a at P30. ( g ) About 11% of striolar Myo7a+ hair cells (HCs) were tdTomato+ at P30. ( h ) Diagram illustrating Type I and II HCs. ( i ) Representative confocal images of P30 damaged and lineage-traced utricles, which contained tdTomato+/Myo7a+ cells with actin-enriched, bundle-like structures. ( i′ – i″ ) Lineage-traced HCs with long (arrowheads) and short stereocilia (arrow). ( j – j″ ) Lineage-traced HCs showed long ( j ), and short ( j′ ) espin+ stereocilia or were espin negative and bundleless ( j″ , labelled by asterisks). ( k ) All tdTomato+/Myo7a+ cells examined expressed Ctbp2 on the basolateral surfaces. k′ shows an orthogonal view of k . ( l ) Lineage-traced HCs were also juxtaposed to the postsynaptic protein Shank1. l′ shows an orthogonal view of l . ( m – m′ ) 92.8% of lineage-traced HCs were innervated by Tuj1+ neurites (arrowhead), a subset of which formed calyces (arrows). ( n ) Lineage-traced HCs were calbindin negative (arrow) and positive (arrowhead). ( o – o′ ) Lineage-traced, Myo7a+ HCs were Sox2 positive (arrowheads) and negative (arrows). ( p ) Quantification of lineage-traced HCs showed that about half were Sox2 negative ( n =28 cells from 3 organs), calbindin positive ( n =47 cells from 3 organs) and surrounded by Tuj1+ calyces (asterisk) ( n =37 cells from 3 organs). n =4–5 at P5, 26–28 in f , g . Data are shown as mean±s.d. ** P <0.01, Student’s t -tests. Scale bars, ( b – e ) 100 μm; ( c′ – e′ , i , m – o ) 20 μm; ( k ) 10 μm; ( i – j″ , l ) 5 μm. Full size image Because we had seen a partial recovery of HC number at P30 using this in vivo damage paradigm, we extended the tracing period to this age and found a significant increase in tdTomato+/Myo7a+ cells in the striolar region ( P <0.0001, Student’s t -test, Fig. 5d–f , Supplementary Table 4 ), suggesting that some Lgr5+ cells gave rise to Myo7a+ HCs. At P5, Myo7a+ cells were rarely tdTomato positive (0.2±0.3%, n =850 cells from 5 organs), whereas 10.7±2.5% expressed tdTomato at P30 ( n =3,523 cells from 28 organs), indicating that a significant proportion of newly generated HCs derived from Lgr5+ cells ( Fig. 5g ). Among all tdTomato+ cells, the proportion that was also Myo7a+ increased from 3.1±4.5% at P5 ( n =53 cells from 5 organs) to 60.6±9.1% at P30 ( P <0.0001, Student’s t -tests, n =635 cells from 28 organs, Fig. 5f , Supplementary Table 4 ), suggesting that many lineage-traced cells had converted to HCs in the striola. In undamaged control utricles, there was no significant increase in lineage-traced Myo7a+ cells at P30 ( P =0.32, Student’s t -test; Fig. 5d,f , Supplementary Fig. 4e,f , Supplementary Table 4 ). We also performed lineage tracing using Pou4f3 DTR/+ ; Plp1 CreERT/+ ; Rosa26R tdTomato/+ mice and found a similar increase in lineage-traced Myo7a+ cells in the striolar region between P3 and P30 ( Supplementary Fig. 4j–l,n , Supplementary Table 4 ). These data further indicate that Lgr5+ cells gave rise to new HCs after damage to the postnatal mouse utricle. We next examined whether lineage-traced Myo7a+ cells possess apical features of utricle HCs, including the actin-rich stereocilia bundle and expression of the actin-bundling protein espin [48] . Using these markers, we detected three major morphologic patterns in regenerated HCs lineage-traced from the Lgr5+ lineage: long stereocilia (12.9±7.8%), short stereocilia (72.4±11.5%) or no stereocilia (14.7±10.4%; n =69 HCs from 7 organs; Fig. 5i,j ). To relay sensory information centrally, HCs form synaptic connections with afferent projections from the vestibular ganglia. These synapses contain pre and postsynaptic components comprised of Ctbp2 and Shank1, respectively [49] , [50] . At P30, all Lgr5 lineage-traced Myo7a+ HCs expressed Ctbp2 and Shank1 on their basolateral surfaces ( n =33–35 HCs from 3 organs; Fig. 5k,l ). Immunostaining for Tuj1 also revealed neural elements juxtaposed to most lineage-traced Myo7a+ HCs (92.8±6.7%; n =37 HCs from 3 organs, Fig. 5m ), suggesting that regenerated HCs are neurally integrated. Utricular HCs are subdivided into Type I and II with the former expressing calbindin and encased by afferent calyces on their basolateral surface; HC-IIs lack these elements yet express Sox2 (refs 12 , 14 , 51 ). As a marker of HC-Is, calbindin was expressed in 48.4±6.5% of Myo7a+ HCs traced from the Lgr5+ lineage ( n =47 cells from 3 organs, Fig. 5n,p ), and 45.6±5.1% of lineage-traced HCs exhibited Tuj1+ calyx-like innervation ( n =37 cells from 3 organs, Fig. 5m,p ). Conversely, 53.7±3.2% lineage-traced HCs were immuno-positive for Sox2 ( n =28 cells from 3 organs, Fig. 5o,p ). In sum, these results show that damage-recruited Lgr5+ cells can give rise to bundle-bearing, neurally connected HCs of both Type I and II. Distinct SC populations contribute to HC regeneration We observed an increase in HC number in both the striolar and extrastriolar regions in the utricles of DT-treated Pou4f3-DTR mice at P30. However, Lgr5+ SCs almost exclusively contributed to regeneration of striolar HCs. Therefore, we hypothesized that Lgr5-negative SCs may act as HC precursors in the extrastriolar domain. Since prior studies have shown that tamoxifen preferentially activates Cre recombinase in extrastriolar SCs in Plp1-CreERT mice [42] , [52] , we employed Plp1 CreERT/+ ; Rosa26R tdTomato/+ mice to test this hypothesis. Tamoxifen (0.75 mg g −1 gavage) administration at P1 induced tdTomato labelling of Sox2+, Myo7a-negative SCs in the striolar and extrastriolar regions 2 days later ( Fig. 6b , Supplementary Fig. 4i ). Using Pou4f3 +/+ ; Plp1 CreERT/+ ; Rosa26R tdTomato/+ littermates as undamaged controls, we examined whether Plp1-Cre+ SCs also contribute to extrastriolar HC regeneration using Pou4f3 DTR/+ ; Plp1 CreERT/+ ; Rosa26R tdTomato/+ mice. After tamoxifen administration at P1, DT treatment (8 h later) similarly led to HC loss and sensory epithelium shrinkage at P7 and subsequent HC regeneration at P30 ( Fig. 6a , Supplementary Fig. 4j–l ). In comparison to undamaged controls, significantly more Myo7a+ HCs were tdTomato+ in the extrastriolar region at P30 (81.1±1.8% and 22.7±4.3%, respectively, P <0.0001, Student’s t -test, Fig. 6b–g , Supplementary Table 4 ). These data show that Plp1+ SCs contribute to HC regeneration in the extrastriolar region after in vivo HC ablation. Figure 6: Striolar and extrastriolar supporting cells behave differently after damage. ( a ) Schematic depicting the use of transgenic mice to ablate hair cells (HCs) and fate-map Plp1+ supporting cells (SCs). ( b , c ) Tamoxifen led to tdTomato labelling of extrastriolar SCs at P3 (also see Supplementary Fig. 4 ). ( d – f ) In both P7 undamaged (not shown) and damaged organs, a subset of Myo7a+ HCs were tdTomato+ (asterisks). Most extrastriolar HCs were tdTomato+ in the P30 damaged utricles, whereas only a subset of HCs were tdTomato+ in the P30 undamaged controls ( f ). ( g ) Quantification showed that damaged organs had significantly more lineage-traced HCs than undamaged controls in the extrastriolar region at P7 and P30 ( n =520–1,884 cells from 4–6 organs). ( h ) In the striolar region where Lgr5 was expressed after damage, significantly more HCs derived from the Lgr5+ than Plp1+ lineage ( n =635 from 28 organs and 1,232 cells from 4 organs, respectively). ( i ) Schematic showing the use of transgenic mice to ablate HCs and fate-map Lgr5+ striolar SCs, and EdU to trace dividing cells. ( j–m ) Undamaged utricles contained few EdU-labelled cells in the sensory epithelium. Damage caused robust EdU labelling in the striolar region, where lineage-traced Lgr5+ cells resided. At P7, most EdU+ cells were Myo7a negative and resided in the SC layer, including EdU+, lineage-traced cells (arrowheads). At P30, many EdU+/tdTomato+/Myo7a+ HCs (arrowheads) were present. ( m′′′ ) Many EdU+/tdTomato+/Myo7a-negative SCs were also found at P30 (arrows). ( m′′′′ ) shows an orthogonal view of m′ ( n =602 cells from 6 organs). ( n ) Quantification of EdU labelling showed that the Lgr5+ lineage (Myo7a-negative SCs in ( m′′′ ) was more proliferative than Sox2+ SCs in the striolar and extrastriolar regions (see Supplementary Fig. 5c,e ). n =4–8 in g and n , and 4–28 in h (4–8 for P3–5, 28 for Lgr5-traced P30 organs and 4–6 for Plp1-traced P30 organs). Data shown as mean±s.d. * P <0.05, ** P <0.01, Student’s t -tests. Scale bars, ( b – f , j – m ) 100 μm; ( k′ , k″ , m′ , m′′′ ) 20 μm. Full size image To determine if Lgr5+ cells are more likely to regenerate HCs than Plp1+ cells in the striolar region, we analyzed utricles from P30 transgenic mice used to trace both lineages. Despite the reported low Cre activity in the striola of Plp1-CreERT mice [42] , we observed many Plp1 lineage-traced SCs using the Rosa26R-tdTomato Cre reporter mice ( Supplementary Fig. 4i ). Because our tracing schemes led to significantly more tdTomato+ cells in the Plp1+ than in Lgr5+ lineages, we measured regenerative capacity as the percentage of tdTomato+ lineage-traced cells that were Myo7a+. In the striolar region where Lgr5 expression was robust ( Fig. 4n ), significantly more tdTomato+ cells of the Lgr5+ lineage than those of the Plp1+ lineage expressed Myo7a at P30 (60.6±9.1% versus 25.7±2.7%, P <0.0001, Student’s t -test, Fig. 6h , Supplementary Table 4 ). In contrast, the extrastriolar region lacked Lgr5 expression and harboured traced Myo7a+ cells from the Plp1+ lineage and not the Lgr5+ lineage ( Fig. 6e , Supplementary Fig. 4g ). These results suggest a spatial segregation of HC progenitors in which a higher proportion of Lgr5+ SCs, compared with Plp1+ SCs, converted to HCs in the striola. Lgr5+ supporting cells proliferate and differentiate into HCs We next asked whether Lgr5+ SCs are more proliferative than Lgr5-negative SCs in response to HC loss. Prior studies demonstrated some proliferative regeneration of HCs in the neonatal mouse utricle [16] . We first marked proliferative cells by administering the mitotic marker EdU (50 mg kg −1 once daily at P4–6) after DT-mediated HC ablation in P1 Pou4f3 DTR/+ mice ( Supplementary Fig. 5a ). At P7 and P30, sensory epithelium in damaged organs had robust EdU labelling, which was rare in undamaged, age-matched controls (wild-type littermates identically injected with DT and EdU, Supplementary Fig. 5b–e ). In undamaged controls, most EdU-labelled cells resided in the stromal layer below the sensory epithelium ( Supplementary Fig. 5b,d ). In damaged organs, significantly more EdU+/Sox2+ SCs resided in the striolar than extrastriolar regions at P7 and P30 ( P <0.0001, Student’s t -tests, for both, Fig. 6n , Supplementary Fig. 5c,e ). Similarly, the striolar region contained more EdU+/Myo7a+ HCs than the extrastriolar region at P7 and P30 ( Supplementary Fig. 5c,e ). Thus, the Lgr5-containing striolar region is significantly more proliferative than the extrastriolar region. To determine the identity of these proliferative cells, we immunostained utricles from P4 Pou4f3 DTR/+ ; Lgr5 EGFP-CreERT2/+ mice and found that 8.1±3.5% Lgr5+ cells expressed the proliferative marker Ki67 ( Supplementary Fig. 6f and Supplementary Table 6 ). Next, we investigated the fate of these damage-activated proliferative cells by combining lineage and mitotic tracing in Pou4f3 DTR/+ ; Lgr5 EGFP-CreERT2/+ ; Rosa26R tdTomato/+ mice (DT at P1, tamoxifen at P3, EdU at P4–6 with Pou4f3 +/+ ; Lgr5 EGFP-CreERT2/+ ; Rosa26R tdTomato/+ mice as controls ( Fig. 6i ). EdU labelled a significantly higher percentage of SCs of the Lgr5 lineage (tdTomato+) than of Sox2+ SCs in the striolar and extrastriolar regions at P7 and P30 ( Fig. 6k,m,n , Supplementary Fig. 5c,e ). At P7, 5.9±2.6% of Myo7a+ HCs were tdTomato labelled, but no EdU+/tdTomato+/Myo7a+ HCs were observed ( n =602 cells from 6 organs, Fig. 6k ). At P30, 22.8±9.8% of tdTomato+/Myo7a+ HCs were EdU labelled ( n =60 cells from 6 organs, Fig. 6m,n ). These results indicate that Lgr5+ cells represent spatially specified HC progenitors that are capable of mitotic HC regeneration in vivo . ß-catenin stabilization promotes proliferation of damage-activated Lgr5+ supporting cells in vivo As the central mediator of canonical Wnt signalling, ß-catenin overexpression has been shown to exert contrasting effects on SCs in the developing cochlea [36] , [37] . We examined the roles of Wnt/ß-catenin signalling on damaged-recruited Lgr5+ cells by generating the Pou4f3 DTR/+ ; Lgr5 EGFP-CreERT2/+ ; Catnb flox(exon3)/+ mice [53] . In this set of experiments, DT was administered at P1 to ablate HCs, tamoxifen (0.075 mg g −1 ) was given at P3 to activate Cre recombinase in Lgr5+ cells and EdU (25 mg kg −1 daily at P4–6) was used to label proliferating cells. Utricles were examined at P30 ( Fig. 7a ). In comparison to DT-damaged utricles without stabilized ß-catenin, damaged organs with stabilized ß-catenin contained larger sensory epithelia (46.2±15.6% and 64.7±4.9% of undamaged controls, respectively, Fig. 7d–f ). In the striolar region where most EdU+ HCs and SCs resided, ß-catenin stabilization caused a modest but significant increase in HCs ( P <0.005, Student’s t -test, Fig. 7d′–e′ ) but not SCs. In addition, activating Wnt signalling in Lgr5+ cells significantly increased both the numbers of EdU+/Myo7a+ cells and EdU+ SCs in the striola ( Fig. 7d′–e″ ) while those in the extrastriola were comparable to DT-damaged organs ( Supplementary Table 5 ). Without DT-mediated damage, tamoxifen did not increase EdU uptake in Lgr5 EGFP-CreERT2/+ ; Catnb flox(exon3)/+ utricles ( Fig. 7b,c,h,i ), suggesting that Lgr5 was not expressed and Cre recombinase activity was absent. Together, these results implicate that ß-catenin stabilization stimulates proliferation and mitotic HC regeneration by damage-activated Lgr5+ SCs. 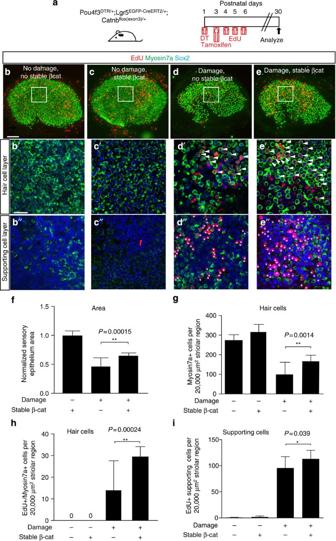Figure 7: Stabilizedß-catenin drives mitotic hair cell regeneration by Lgr5+ cells. (a) Schematic of usingPou4f3DTR/+;Lgr5EGFP-CreERT2/+;Catnbflox(exon3)/+mice to express stabilized ß-catenin in Lgr5+ cells after hair cell ablation. EdU was administered to label proliferating cells. (b) Undamaged, controls showed almost no EdU labelling in the sensory epithelium. (c) Utricles fromLgr5EGFP-CreERT2/+;Catnbflox(exon3)/+mice treated with tamoxifen also showed no increased EdU uptake. (d) Damage utricles showed fewer Myo7a+ hair cells (HCs) and increased EdU+ HCs and supporting cells (SCs) in the striolar region. (e) Stabilized ß-catenin in Lgr5+ cells enhanced HC density and EdU labelling of HCs and SCs in the striolar region. (f,g) Sensory epithelium size and HC density significantly increased after ß-catenin stabilization in Lgr5+ cells. (h,i) Relative to damage alone, ß-catenin stabilization in Lgr5+ cells significantly increased the number of EdU+/Myo7a+ HCs and EdU+ SCs in the striolar region.n=5–18 inf–i(18 for damaged organs without ß-catenin stabilization, 5–8 for all other groups). Data are shown as mean±s.d. *P<0.05, **P<0.01, Student’st-tests. Scale bars, (b–e) 100 μm; (b′–e″) 20 μm. Figure 7: Stabilized ß -catenin drives mitotic hair cell regeneration by Lgr5+ cells. ( a ) Schematic of using Pou4f3 DTR/+ ; Lgr5 EGFP-CreERT2/+ ; Catnb flox(exon3)/+ mice to express stabilized ß-catenin in Lgr5+ cells after hair cell ablation. EdU was administered to label proliferating cells. ( b ) Undamaged, controls showed almost no EdU labelling in the sensory epithelium. ( c ) Utricles from Lgr5 EGFP-CreERT2/+ ; Catnb flox(exon3)/+ mice treated with tamoxifen also showed no increased EdU uptake. ( d ) Damage utricles showed fewer Myo7a+ hair cells (HCs) and increased EdU+ HCs and supporting cells (SCs) in the striolar region. ( e ) Stabilized ß-catenin in Lgr5+ cells enhanced HC density and EdU labelling of HCs and SCs in the striolar region. ( f , g ) Sensory epithelium size and HC density significantly increased after ß-catenin stabilization in Lgr5+ cells. ( h , i ) Relative to damage alone, ß-catenin stabilization in Lgr5+ cells significantly increased the number of EdU+/Myo7a+ HCs and EdU+ SCs in the striolar region. n =5–18 in f – i (18 for damaged organs without ß-catenin stabilization, 5–8 for all other groups). Data are shown as mean±s.d. * P <0.05, ** P <0.01, Student’s t -tests. Scale bars, ( b – e ) 100 μm; ( b′ – e″ ) 20 μm. Full size image Hearing and balance functions require mechanosensory HCs, and diseases that cause HC degeneration manifest as hearing or balance disorders. In the mature mammalian cochlea, the absence of HC regeneration underlies the permanence of hearing loss [54] , [55] . The mammalian vestibular epithelium, however, exhibits a limited regenerative capacity and therefore serves a useful preparation to examine mammalian HC regeneration. Here we have identified Lgr5+ cells as region-specific HC progenitors capable of both mitotic and non-mitotic HC regeneration at early postnatal stages. Moreover, we show that Wnt/ß-catenin signalling can modestly enhance mitotic regeneration by Lgr5+ cells in the damaged neonatal utricle. While utricular HCs are functional in the neonatal period [56] , [57] , prior studies comparing neonatal to adult utricles found differences in cellular composition [12] , [42] , responsiveness to Notch inhibition [18] , [58] and proliferative responses to damage [16] , [23] . Specifically, the neonatal utricle can proliferate and mitotically regenerate HCs, whereas the primary mode of HC regeneration in the adult organ is direct transdifferentiation. Because both modes of HC regeneration operate in non-mammalian vertebrates to restore auditory and vestibular functions, they are likely important in restoring the proper cytoarchitecture and functions of HCs and SCs [7] , [59] . Our data indicate that Lgr5+ cells in the neonatal utricle are capable of regenerating HCs via both direct transdifferentiation and mitotic regeneration. Moreover, in the adult utricle, HC regeneration is mainly in the extrastriolar region in which regenerated HCs are primarily Type II (refs 17 , 23 ). While both HC-Is and HC-IIs function as mechanoreceptors, the former are concentrated in the striolar region, and they are morphologically and functionally distinct from HC-IIs [12] . Our study shows that Lgr5+ cells in the neonatal utricle can regenerate both HC-Is and HC-IIs, behaviour that is reminiscent of SCs from avian utricles in which both types of HCs are spontaneously regenerated [7] . Therefore, future studies defining the molecular signatures of Lgr5+ cells may help reveal factors regulating the regeneration of distinct HC subtypes and also those dictating the two modes of HC regeneration. As HCs are still being born with committed HCs maturing, SCs in the neonatal utricle may be less mature and more plastic than those in the adult organ, possibly accounting for their differential responses to damage. In addition, it is important to note that while Lgr5 expression was induced by damage both in vitro and in vivo , behaviour of Lgr5+ cells in the two systems differ in that direct transdifferentiation predominated and mitotic regeneration was absent in vitro , and the degree of HC regeneration was much less robust than that observed in vivo ( Supplementary Fig. 6 and Supplementary Table 6 ). After neomycin damage in vitro (14DIV), 19.3±5.0 striolar HCs per organ were fate-mapped from the Lgr5 lineage. One month after HC ablation in vivo , 38.7±6.2 Lgr5 lineage-traced HCs were noted in the striola of each organ. We postulate that the different damage models used (neomycin in vitro versus diphtheria toxin in vivo ) may have, at least in part, caused these differences by inflicting more damage in vitro as degenerating Lgr5+ SCs (which appeared smaller, TUNEL positive and Sox2 negative) were more frequently observed in vitro than in vivo . As a result, the persistence of Lgr5 expression observed in vitro (and not in vivo ) may reflect an undifferentiated state [1] , [30] , in which damaged-recruited Lgr5+ cells lack additional cues that are required for them to proliferate and/or differentiate. To add to this complexity, the culture system may also lack secreted mitogenic/prosensory factors normally present in vivo , with candidates including TGFα, EGF and possibly other family members [60] , [61] . Thus future studies comparing the in vitro and in vivo systems may shed light on factors limiting or driving spontaneous HC regeneration in mammals. Canonical Wnt signalling becomes activated after damage and mediates repair in multiple organ systems [4] , [30] , [32] . In the current study, embryonic Lgr5+ cells contributed to otherwise quiescent resident cells that became recruited in response to tissue injury. Similarly in the mammary gland, Wnt-responsive cells contribute to organ development as well as to the resident progenitor cells that are recruited for glandular outgrowth during pregnancy [62] . In less regenerative organs such as the liver and pancreas, tissue damage similarly elicits the emergence of Lgr5+ progenitors cells, which can be expanded in vitro in a Wnt-dependent manner to form organoids consisting of mature cell types [30] , [31] . Overactive Wnt signalling can also induce pathologic states as a result of uncontrolled proliferation and a lack of cellular differentiation [34] , [35] . In the developing cochlea, conflicting results have been observed as a result of ß-catenin stabilization [36] , [37] . Our data indicate that ß-catenin stabilization resulted in a modest increase in HC density and more remarkably the number of EdU-labelled HCs and SCs, suggesting that canonical Wnt signalling primarily serves as a proliferative signal to Lgr5+ cells but does not limit their HC fate ( Fig. 8 ). These results lead us to propose that other instructive signals, possibly including increased Atoh1 expression and decreased Notch signalling [18] , [63] , [64] , [65] , [66] , [67] , can be complementary for driving HC regeneration. While active Wnt signalling may be used to increase the population of competent cells, more work is necessary to test the feasibility and success of such combinatorial approaches. 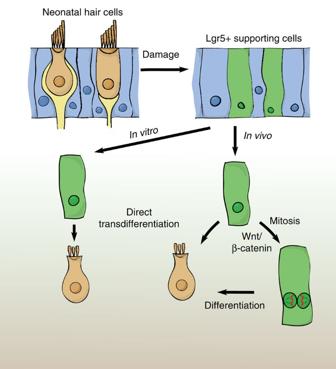Figure 8: Model of hair cell regeneration in the neonatal mouse utricle. Striolar supporting cells (SCs) expressLgr5after hair cell (HC) ablationin vitroandin vivo(16.8% and 28.5%, respectively). After neomycin-induced HC loss, Lgr5+ SCs regenerate HCs via direct transdifferentiationin vitro. After HC ablationin vivo, Lgr5+ SCs regenerate HCs using both mitotic and non-mitotic mechanisms. Activating Wnt signalling promotes mitotic HC regeneration. Figure 8: Model of hair cell regeneration in the neonatal mouse utricle. Striolar supporting cells (SCs) express Lgr5 after hair cell (HC) ablation in vitro and in vivo (16.8% and 28.5%, respectively). After neomycin-induced HC loss, Lgr5+ SCs regenerate HCs via direct transdifferentiation in vitro . After HC ablation in vivo , Lgr5+ SCs regenerate HCs using both mitotic and non-mitotic mechanisms. Activating Wnt signalling promotes mitotic HC regeneration. Full size image In summary, we report that HC loss results in induction of Lgr5 in a subset of striolar SCs, which can behave as facultative HC progenitors in the neonatal utricle in vitro and in vivo . Therefore, Lgr5+ cells may be useful for further dissecting the mechanisms governing mammalian HC regeneration. Mice Lgr5 –EGFP -CreERT2 (Jackson Laboratory, #8875) [1] , Plp1-CreERT (Jackson Laboratory, #5975) [68] , Rosa26R-tdTomato (Jackson Laboratory, #7908) [41] , Pou4f3-DTR [23] and Catnb-flox(exon3) [53] mice of both genders were used. For Cre activation, tamoxifen (dissolved in corn oil; Sigma) was given via gavage to neonatal mice (0.075 mg g −1 for Lgr5 –EGFP -CreERT2 and 0.75 mg g −1 Plp1-CreERT strains) and dams (0.225 mg g −1 , i.p.). Diphtheria toxin (6.25 ng g −1 i.p., List Biological Laboratories) and EdU (25–50 mg kg −1 i.p., Invitrogen) were used. All protocols were approved by Animal Care and Use Committee of the Stanford University School of Medicine, St. Jude Children’s Research Hospital and NIH. Cell quantification and statistics Cells were quantified from z-stack images of 20,000 μm 2 using Volocity software (v6.1.0; Improvision) unless otherwise stated. Images were taken from 1–2 representative areas from the striolar (each area is ∼ 20,000 μm 2 and represent 35–48% of the striola, which we defined as oncomodulin+, Lgr5+ or Lgr5 lineage-traced domains, see Fig. 4f′ , Supplementary Fig. 1a , Supplementary Table 2 for details) or extrastriolar regions for analyses. In damaged tissues where oncomodulin-marked HC-I had degenerated, Lgr5 or Lgr5 lineage-traced expression was used to define the striolar region. For all experiments, n values represent the number of cells or organs examined unless otherwise stated. Statistical analyses were conducted using Microsoft Excel (Microsoft) and GraphPad Prism 5.0 software (GraphPad). Two-tailed, unpaired Student’s t -tests were used to determine statistical significance. P <0.05 was considered as significant. Data are shown as mean±s.d. Whole organ cultures Utricles were harvested from E19.5-P5 mice of both genders and otoconia removed in sterile conditions, and then attached to coverslips (10 mm, Marienfeld) pre-coated with CellTaK (BD Biosciences) and placed in four-well Petri dishes (CellStar). Whole organs were cultured in growth factor-enriched, serum-free media, consisting of DMEM/F12 (1:1; Cellgro), N2 (1:100), B27 (1:50, both from Invitrogen), bFGF (1 ng ml −1 ), IGF-1 (50 ng ml −1 ), EGF (20 ng ml −1 ), heparin sulfate (50 ng ml −1 ) and ampicillin (50 ng ml −1 ; all from Sigma). The following agents were added to a subset of cultures: neomycin (1.0 mM, Sigma), EdU (1.0 μM), 4OH-tamoxifen (500 nM, Sigma). Genotyping and real time quantitative PCR Standard PCR was performed to genotype transgenic mice using genomic DNA. DNA was isolated by adding 200 μl of 50 mM NaOH to cut tail tips, incubating at 98 °C for 1 h, and then adding 20 μl of 1 M Tris-HCl. For quantitative PCR (qPCR), total RNA was isolated with RNeasy mini extraction kits (Qiagen), then complementary DNA was synthesized using SuperScript III First-Strand Synthesis System kits (Invitrogen). SYBR Green PCR Mix kit (Applied Biosystems) was used to perform qPCR reactions on a 7900HT-Fast Real time PCR system (Applied Biosystems). All qPCR reactions were performed in triplicate and relative quantification of gene expression was analyzed using the ΔΔCT method with GAPDH as the endogenous reference [69] . Primers used are listed in Supplementary Table 7 . Immunohistochemistry Utricles were fixed for 1 h in 4% paraformaldehyde (in PBS, pH 7.4; Electron Microscopy Services) at room temperature. [70] Tissues were blocked with 5% goat or donkey serum, 0.1% Triton-X100, 1% bovine serum albumin (BSA), and 0.02% sodium azide (NaN3) in PBS at pH 7.4 for 1–2 h at room temperature, followed by incubation with primary antibodies diluted in the same blocking solution overnight at 4 °C in a humidified chamber. The next day, after washing with PBS, tissues were incubated with secondary antibodies diluted in 0.1% Triton-X100, 0.1% BSA and 0.02% NaN3 solution in PBS for 1 h at room temperature. After PBS washing, tissues were then mounted in antifade Fluorescence Mounting Medium (DAKO) and coverslipped. We used antibodies against the following markers: Myosin7a (1:1,000; Proteus Bioscience or Labome), Tuj1 (1:1,000; Neuromics), Ki67 (1:1,000; Abcam), Gfi1 (1:1,000; gift from H. Bellen), Calbindin (1:1,000; Millipore), Espin (1:1,000, gift from S. Heller), Ctbp2 (1:100; BD Transduction Laboratories), Shank1 (1:100; Neuromics), Sox2 (1:400), Jag1 (1:200), and Oncomodulin (1:250, all from Santa Cruz Biotechnology). The secondary antibodies were conjugated with FITC, TRITC or Cy5 (1:500, Invitrogen). Fluorescent-conjugated phalloidin (1:1,000; Sigma), DAPI (1:10,000; Invitrogen) and Alexa Fluor 488, 555 or 647 EdU detection kit (Invitrogen) were used. TUNEL Alexa Fluor 594 imaging Assay kit (Invitrogen) was used in accordance to kit instructions. Images were acquired using epifluorescent or confocal microscopy (Axioplan 2, Zeiss Pascal or LSM700) and analyzed with Image J64 (NIH) and Photoshop CS4 (Adobe Systems). Three-dimensional reconstruction of z-stack images was performed with Volocity software. In situ hybridization In situ hybridization was performed on cultured P3 wild-type utricles using RNAscope probes for Lgr5 according to manufacturer’s instructions (Advanced Cell Diagnostics). Probes for DapB were used as negative controls. Utricles were fixed for 1.5 h in 4% paraformaldehyde and washed in PBS before being hybridized with probes for 2 h at 40 °C. Signal was amplified and detected with 2.0 HD reagent Kit-RED and imaged on the EVOS XL Core Imaging system (Life Technologies). Time-lapse imaging Utricles harvested from P3–P5 Lgr5 EGFP-CreERT2/+ ; Rosa26R tdTomato/+ mice were attached to 35 mm glass bottom dishes (MatTek) pre-coated with CellTaK. Whole organs were cultured overnight, then treated with neomycin (1.0 mM × 24 h, Sigma) as above. 4OH-tamoxifen (500 nM, Sigma) in growth factor-enriched, serum-free media was present for 2–4 days first. Then organs were imaged in DMEF/F12 without phenol red media using a spinning disc confocal imaging system (Zeiss Axio Observer Z1 or OlympusIX-81 coupled with a Yokogawa spinning disc system CSU-X1A 5000) connected to an incubating chamber (37 °C, 5% CO 2 ). One to two EGFP+ regions with tdTomato+ cells were selected from each utricle, and z-stack images spanning the sensory epithelium were taken at 0.5–1 h intervals. Collected videos were processed and analyzed with Image J64, MetaMorph (NX 2.0; Olympus) and Volocity software. How to cite this article: Wang, T. et al. Lgr5+ cells regenerate hair cells via proliferation and direct transdifferentiation in damaged neonatal mouse utricle. Nat. Commun. 6:6613 doi: 10.1038/ncomms7613 (2015).